Mechanistic evaluation and transcriptional signature of a glutathioneS-transferase omega 1 inhibitor Glutathione S -transferase omega 1 (GSTO1) is an atypical GST isoform that is overexpressed in several cancers and has been implicated in drug resistance. Currently, no small-molecule drug targeting GSTO1 is under clinical development. Here we show that silencing of GSTO1 with siRNA significantly impairs cancer cell viability, validating GSTO1 as a potential new target in oncology. We report on the development and characterization of a series of chloroacetamide-containing potent GSTO1 inhibitors. Co-crystal structures of GSTO1 with our inhibitors demonstrate covalent binding to the active site cysteine. These potent GSTO1 inhibitors suppress cancer cell growth, enhance the cytotoxic effects of cisplatin and inhibit tumour growth in colon cancer models as single agent. Bru-seq-based transcription profiling unravelled novel roles for GSTO1 in cholesterol metabolism, oxidative and endoplasmic stress responses, cytoskeleton and cell migration. Our findings demonstrate the therapeutic utility of GSTO1 inhibitors as anticancer agents and identify the novel cellular pathways under GSTO1 regulation in colorectal cancer. Glutathione S -transferases (GSTs) are a diverse family of cytosolic, mitochondrial and microsomal enzymes that are primarily involved in phase II metabolism. In addition to xenobiotic detoxification through glutathione conjugation, GSTs also play a key role in the synthesis and metabolism of endogenous compounds, redox homeostasis and cellular signalling [1] , [2] . GST overexpression and polymorphisms are seen in several cancers as well as other diseases, and have been implicated in resistance to chemotherapy [2] , [3] . Thus, they are attractive anticancer targets. Indeed, several small-molecule GST inhibitors have been reported as anticancer agents [4] . The mammalian cytosolic GSTs are classified into seven different classes—alpha, mu, pi, theta, sigma, zeta and omega. Among them, the omega GSTs (GSTO) belong to an atypical cytosolic class. They share low sequence identity with other GST classes, but still exhibit the characteristic GST fold [5] , [6] . GSTOs have a cysteine residue at the catalytic site in place of the characteristic tyrosine or serine. Consequently, instead of glutathione conjugation, GSTOs catalyse thioltransferase reactions similar to glutaredoxins. In humans, two GSTO isozymes GSTO1 and GSTO2 have been identified. They share 64% sequence identity and differ in their catalytic activities. GSTO1 catalyses S -phenacyl glutathione reduction and monomethylarsonate (V) reduction, while GSTO2 has a prominent dehydroascorbate reductase activity [7] . The cellular functions of GSTO1 have not been fully elucidated, although a role in cellular stress responses is emerging [8] , [9] , [10] . Recently, a significant role for GSTO1 in protein deglutathionylation has been described [11] , and β-actin was identified as one of the cellular substrates for GSTO1-catalysed deglutathionylation. Studies have also proposed a role in ryanodine receptor modulation, interleukin-1β (IL-1β) secretion and endoplasmic reticulum stress-mediated autophagy [7] , [12] , [13] , [14] , [15] . Interestingly, GSTO1 polymorphisms and decreased expression have been implicated in several pathological conditions such as Parkinson’s and Alzheimer’s disease [7] . In addition, GSTO1 overexpression has been documented in breast cancer cell lines [16] , [17] and has a role in the development of drug resistance [7] , [18] , [19] . Thus, GSTO1 is an attractive pharmacological target, for which, there is a need for potent and selective inhibitors. Small molecules and peptides bearing electrophilic moieties have previously been reported as GSTO1 inhibitors [20] , [21] , [22] , [23] , [24] . In particular, compounds containing α-chloroacetamide moieties have shown potent inhibitory activity. However, characterization of their effects in cancer cells is limited. Here we report on the development and characterization of small-molecule inhibitors of GSTO1 and the use of these inhibitors to study the cellular functions of GSTO1. We have identified a family of chloroacetamide-containing compounds with potent inhibitory activity against GSTO1 and efficacy against cancer cells in both in vitro and in vivo models. In addition, these compounds inhibited IL-1β secretion from monocytic cells. We further show using siRNA that GSTO1 is an important survival factor for cancer cells. Through transcriptional profiling using Bru-seq, we also uncover novel cellular pathways regulated by GSTO1. Taken together, our findings validate GSTO1 as an important drug target for cancer therapeutics. Importantly, we have solved the crystal structure of our potent inhibitors in complex with GSTO1, paving the way for rational design of optimized GSTO1 inhibitors. Identification of C1-27 as a potent GSTO1 inhibitor The α-chloroacetamide is a privileged scaffold that has been commonly used to target cysteine residues on various proteins [20] , [21] , [25] . We synthesized a set of novel small molecules based on a 2-chloro- N -phenylacetamide scaffold, evaluated their effects on GSTO1 activity and explored structure–activity relationships ( Supplementary Fig. 1 ). For activity screening, we adapted a GSTO1 substrate assay that relies on the quantification of the reduction of S -(4-nitrophenacyl)glutathione (4-NPG), a GSTO1-specific substrate [17] , using recombinant human GSTO1 in a high-throughput screening format. The Z ′ factor value for the assay was 0.73 ( Supplementary Fig. 2 ). 4a , one of the initial hits, inhibited GSTO1 enzyme activity with a half-maximal inhibitory concentration (IC 50 ) value of 3.1 μM. 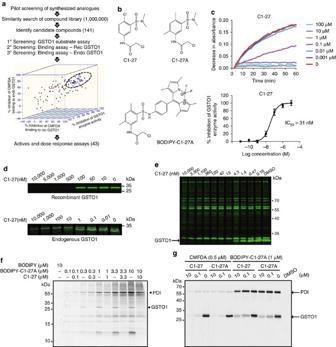Figure 1: Identification and characterization of C1-27 as a potent GSTO1 inhibitor. (a) Schematic of small-molecule screening and inhibitor identification. (b) Chemical structures of lead inhibitorC1-27, related analogueC1-27Aand BODIPY-conjugatedC1-27A. (c)C1-27significantly inhibited GSTO1-catalysed 4-nitrophenacyl glutathione reduction in a dose-dependent manner. (Below) Plot shows % inhibition of GSTO1 activity byC1-27, calculated from absorbance values atT=30 min. Curves generated from mean values of five independent experiments (error bars, s.e.m.). (d)C1-27potently competes with CMFDA for binding to recombinant GSTO1 (top) and endogenous GSTO1 in HCT116 soluble proteome (bottom). Competitive inhibition of CMFDA binding was assessed by in-gel fluorescence scanning. One of three independent experiments is shown. (e)C1-27competes with CMFDA for binding to GSTO1 without affecting labelling of other proteins, demonstrated by in-gel fluorescence binding assay. One of three independent experiments is shown. (f) Fluorescence scan of proteins labelled by BODIPY-C1-27Ain HCT116 cells in the presence and absence of pretreatment withC1-27at indicated concentrations. Representative image of two independent experiments is shown in greyscale for clarity. Arrows indicate bands corresponding to GSTO1 and PDI. (g)C1-27orC1-27Apotently inhibited BODIPY-C1-27Aand CMFDA binding to recombinant GSTO1 while modestly inhibiting PDI labelling. Representative image of two independent experiments is shown. We observed that addition of electron-withdrawing substituents on the phenyl ring increased the electrophilicity of the chloroacetamide carbon and improved potency of inhibition ( Supplementary Table 1 ). We next performed a structural similarity search across our in-house compound collection, as well as on commercial small-molecule libraries ( ∼ 1,000,000 compounds) and identified 141 additional hits, which were screened in the high-throughput activity assay at a single concentration of 10 μM. Their GSTO1 inhibitory activity was further confirmed by a competitive binding assay. Using 5-chloromethylfluorescein diacetate (CMFDA), which has been reported to be a potent and irreversible GSTO1 inhibitor [22] , we optimized a gel-based binding assay that measures competitive inhibition of CMFDA binding to recombinant GSTO1 or endogenous GSTO1 in a soluble proteome ( Supplementary Fig. 3 ). The general approach for inhibitor identification is outlined in Fig. 1a . On the basis of their structures, the hits were grouped into five different clusters ( Supplementary Figs 4–8 ). Among the different clusters, cluster-1, based on a N -phenyl-2°-chloroacetamide scaffold, yielded some of the most potent active compounds. Replacing the phenyl ring with a heterocyclic moiety was also well tolerated and resulted in potent hits (cluster-2). Cluster-3 consisting of N- linker-2°-chloroacetamides was mostly inactive, suggesting that inclusion of additional linker groups between the chloroacetamide moiety and the aromatic centre decreased its electrophilic nature and negatively affected potency. Similarly, replacing the 2°-chloroacetamide with a 3°-chloroacetamide derivative such as in cluster-4 also proved unfavourable and resulted in loss of potency. On the other hand, cyclization of the 3°-chloroacetamide restored activity (cluster-5). From this preliminary screening, we selected 43 compounds that showed at least 50% inhibition in all three assays for further dose–response studies ( Supplementary Tables 2–6 ). Inhibitory profile of selected potent compounds is shown in Supplementary Table 7 . Interestingly, some of the top hits from this large unbiased screen belonged to the N -(3-sulfamoyl)phenyl chloroacetamide class of compounds. Among them, C1-27 was one of the most potent GSTO1 inhibitors ( Fig. 1b ). C1-27 potently inhibited GSTO1 enzyme activity with an IC 50 value of 31 nM ( Fig. 1c ). It also potently competed with CMFDA for binding to recombinant protein, as well as endogenous GSTO1 in the milieu of a soluble proteome ( Fig. 1d ). While the fluorescent dye CMFDA labelled several other cysteine-containing proteins in the proteome, C1-27 showed a selective inhibition of the GSTO1 band up to 1 μM ( Fig. 1e ). To further examine C1-27 selectivity and to detect other possible targets, we synthesized a fluorescent BODIPY conjugate of a C1-27 analogue. Attempts at generating BODIPY-conjugated C1-27 were unsuccessful as it proved to be unstable. Instead, we used C1-27A , a close structural analogue with a similar inhibitory profile ( Fig. 1b and Supplementary Fig. 9 ). Analysis of the HCT116 soluble proteome showed that BODIPY- C1-27A bound GSTO1 even at sub-micromolar concentrations. In addition, BODIPY- C1-27A also strongly labelled a 57 kDa band corresponding to protein disulfide isomerase (PDI), a chaperone protein with cysteine at its active site ( Fig. 1f and Supplementary Fig. 10a ). Compounds containing α-chloroacetamide moieties have been shown to bind PDI [25] . Above 1 μM, BODIPY- C1-27A showed an increased nonspecific reactivity that was not inhibited by pretreatment with unconjugated C1-27A ( Supplementary Fig. 10b ). Similarly, pretreatment with C1-27 selectively blocked BODIPY- C1-27A binding to GSTO1 up to 1 μM. Furthermore, C1-27 bound GSTO1 more potently than PDI and showed a 100-fold more potent inhibition of its enzyme activity ( Fig. 1f,g and Supplementary Table 7 ). In a cellular thermal-shift assay, we observed GSTO1 engagement by C1-27 even at lower concentrations (1 μM), while a thermal shift for PDI was observed only at higher concentrations ( Supplementary Fig. 11 ). Other potent GSTO1 inhibitors also showed a similar selectivity profile ( Supplementary Fig. 10c and Supplementary Table 7 ). These findings suggest that despite bearing a reactive electrophile, C1-27 did not bind to cellular proteins indiscriminately but appeared to exhibit certain degree of selectivity in target binding. Figure 1: Identification and characterization of C1-27 as a potent GSTO1 inhibitor. ( a ) Schematic of small-molecule screening and inhibitor identification. ( b ) Chemical structures of lead inhibitor C1-27 , related analogue C1-27A and BODIPY-conjugated C1-27A . ( c ) C1-27 significantly inhibited GSTO1-catalysed 4-nitrophenacyl glutathione reduction in a dose-dependent manner. (Below) Plot shows % inhibition of GSTO1 activity by C1-27 , calculated from absorbance values at T =30 min. Curves generated from mean values of five independent experiments (error bars, s.e.m.). ( d ) C1-27 potently competes with CMFDA for binding to recombinant GSTO1 (top) and endogenous GSTO1 in HCT116 soluble proteome (bottom). Competitive inhibition of CMFDA binding was assessed by in-gel fluorescence scanning. One of three independent experiments is shown. ( e ) C1-27 competes with CMFDA for binding to GSTO1 without affecting labelling of other proteins, demonstrated by in-gel fluorescence binding assay. One of three independent experiments is shown. ( f ) Fluorescence scan of proteins labelled by BODIPY- C1-27A in HCT116 cells in the presence and absence of pretreatment with C1-27 at indicated concentrations. Representative image of two independent experiments is shown in greyscale for clarity. Arrows indicate bands corresponding to GSTO1 and PDI. ( g ) C1-27 or C1-27A potently inhibited BODIPY- C1-27A and CMFDA binding to recombinant GSTO1 while modestly inhibiting PDI labelling. Representative image of two independent experiments is shown. Full size image Co-crystal structures of inhibitors in complex with GSTO1 We determined the structures of GSTO1 bound to three inhibitors ( C1-27 , C1-31 and C4-10 ) by X-ray crystallography ( Fig. 2a and Supplementary Fig. 12 ). In each case, difference electron density maps contoured at 3 σ show each inhibitor covalently bound to the Sγ atom of C32 in GSTO1 ( Supplementary Fig. 13 ). All three inhibitors bind primarily to the hydrophobic or electrophile binding site (H-site) [5] of GSTO1, but do so in unique ways ( Supplementary Fig. 14 ). C1-31 and C4-10 bind solely through hydrophobic interactions, whereas C1-27 binding incorporates both hydrophobic and hydrophilic interactions. In biochemical assays, C1-27 had the highest affinity for GSTO1, which is supported by the structure in that C1-27 makes more interactions with the protein than the other two inhibitors. 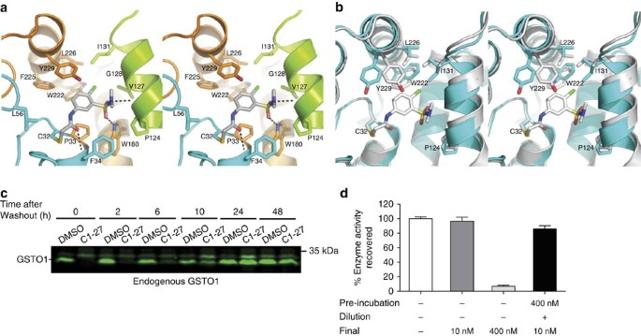Figure 2: C1-27 is a covalent GSTO1 inhibitor. (a) Stereodiagram ofC1-27bound to GSTO1 (PDB ID 4YQM). Ribbon diagram represents the backbone of GSTO1 with residues interacting with the inhibitor shown as ball-and-stick. Residues in cyan contribute to the G-site, while the H-site is made of the residues shown in orange and green (4b helix). The inhibitors are shown in ball-and-stick with carbon atoms in grey, sulfurs in yellow, nitrogens in blue, oxygens in red and chloride in green. The black dashed lines represent hydrogen bonds between the protein and the inhibitor. (b) The crystal structure of GSTO1-C1-27(grey) overlayed onto GSTO1-GSH (cyan) (PDB ID 1EEM) with the residues having the largest change shown in ball-and-stick. The overall root mean squared deviation between the GSTO1-C1-27and 1EEM structures is 0.614 Å. (c) CMFDA labelling of GSTO1 was inhibited byC1-27up to 6 h and recovered completely by 24 h. One of three independent experiments is shown. (d)C1-27acts as a slow-turnover substrate demonstrated by 86% recovery of enzyme activity after pre-incubation and a large dilution in the GSTO1 substrate assay. Experiments were performed in triplicate (error bars, s.e.m.). Figure 2: C1-27 is a covalent GSTO1 inhibitor. ( a ) Stereodiagram of C1-27 bound to GSTO1 (PDB ID 4YQM). Ribbon diagram represents the backbone of GSTO1 with residues interacting with the inhibitor shown as ball-and-stick. Residues in cyan contribute to the G-site, while the H-site is made of the residues shown in orange and green (4b helix). The inhibitors are shown in ball-and-stick with carbon atoms in grey, sulfurs in yellow, nitrogens in blue, oxygens in red and chloride in green. The black dashed lines represent hydrogen bonds between the protein and the inhibitor. ( b ) The crystal structure of GSTO1- C1-27 (grey) overlayed onto GSTO1-GSH (cyan) (PDB ID 1EEM) with the residues having the largest change shown in ball-and-stick. The overall root mean squared deviation between the GSTO1- C1-27 and 1EEM structures is 0.614 Å. ( c ) CMFDA labelling of GSTO1 was inhibited by C1-27 up to 6 h and recovered completely by 24 h. One of three independent experiments is shown. ( d ) C1-27 acts as a slow-turnover substrate demonstrated by 86% recovery of enzyme activity after pre-incubation and a large dilution in the GSTO1 substrate assay. Experiments were performed in triplicate (error bars, s.e.m.). Full size image The structure of the GSTO1– C1-27 complex was solved to 2.4 Å resolution with three molecules per asymmetric unit. The bound C1-27 interacts predominately with residues in the H-site with only three interactions with the glutathione-binding site (G-site) ( Fig. 2a ). The backbone amide nitrogen of F34 from the G-site stabilizes the acetamide oxygen position via a hydrogen bond and the phenyl ring of F34 packs edge on with the phenyl group of C1-27 . The third interaction is between the side chain of L56 (Cδ1) and the carbon atom of the acetamide group. The rest of the atoms within C1-27 interact with the H-site causing rearrangement of several side chains and a 1 Å shift in the 4b helix (residues 122–132) with respect to the GSTO1-GSH structure (1EEM) ( Fig. 2b ). The side chains of W222 and I131 rotate 180° and 90°, respectively, compared with the 1EEM structure due to the binding of the C1-27 chloride atom. The chloride is located in a hydrophobic pocket interacting with I131 Cδ1, V127 Cγ1 and W222 Cζ. The side chain of Y229 also differs from the 1EEM structure, swinging >49° to form a partial π -stacking with the phenyl group of the inhibitor. The entire 4b helix shifts ∼ 1 Å in comparison to the 1EEM structure due to the sulfonamide group interacting with three residues (G128, V127 and P124) within the helix. These residues form hydrophobic interactions with the methyl groups, while the carbonyl O of P124 hydrogen bonds with the nitrogen atom, which conforms to a tetrahedral configuration suggesting that it is protonated. The O2 oxygen of the sulfonamide accepts a hydrogen bond from W180. The other H-site residues (L226, F225 and P33) form van der Waals interactions with the phenyl group of C1-27 . Similar structural rearrangements in W222 and Y229 have been reported with the binding of GSSG in the H-site [26] . The GSTO1– C1-31 structure was determined to 1.94 Å resolution with two molecules in the asymmetric unit ( Supplementary Fig. 12a ). The position of the acetamide group of C1-31 is stabilized by hydrophobic interactions with the side chains of G-site residues L56 and V72. The side chains of F34 and P33 interact with the bottom of the phenyl ring. The seven-membered ring is flanked on three sides by Y229, I131, L226 and F225. The only interaction with the sulfonamide group is V127. The side chains of all residues in the binding site are reminiscent of the 1EEM structure. The GSTO1– C4-10 structure solved to 2.10 Å resolution has two residues (Y229 and W222) that differ from the 1EEM structure. Y229 is positioned in an equivalent manner as in the GSTO1– C1-27 structure, but it does not interact with C4-10 , therefore is not shown in Supplementary Fig. 12b . W222 is rotated and pushed aside to accommodate the phenyl group of C4-10 , which is inserted deeply into the protein surrounded by W222, F225, L226, I131, M187, R183 and V127. The pyrazole group interacts with P33, while the side chains of residues M29 and L56 from the G-site interact with the acetamide group. In line with the covalent binding mechanism, in vitro and cell-based thermal-shift assays showed that C1-27 induced a negative shift in the melting temperature indicating protein destabilization on binding ( Supplementary Figs 11 and 15 ). To further examine the nature of GSTO1–inhibitor complexes, we analysed the time course of GSTO1 labelling by CMFDA following pretreatment of HCT116 cells with C1-27 . GSTO1 labelling was inhibited up to 6 h and then recovered completely by 24 h ( Fig. 2c ). 4a , on the other hand, was more resistant to the washout and inhibited CMFDA labelling up to 24 h ( Supplementary Fig. 16a ). We further examined C1-27 dissociation and GSTO1 reactivation using a pre-incubation and dilution assay. Recombinant GSTO1 was pre-incubated with C1-27 at 400 nM, followed by a 40-fold dilution into assay buffer to a final concentration of 10 nM. Interestingly, 86% of GSTO1 activity was recovered ( Fig. 2d ), suggesting that C1-27 acts as a slow-turnover substrate. Other close analogues of C1-27 also showed a similar regeneration of GSTO1 activity on dilution ( Supplementary Fig. 16d ). The mechanism of enzyme regeneration is unclear, although we speculate that presence of a reducing agent such as dithiothreitol (DTT) in the assay buffer could facilitate the recovery. In contrast, enzyme activity following 4a incubation was not recovered on dilution, indicating an irreversible covalent bond with the enzyme ( Supplementary Fig. 16c ). GSTO1 inhibition is cytotoxic to cancer cells We evaluated the expression of GSTO1 in various tumour types using publicly available gene expression data sets from the Oncomine database. GSTO1 was significantly overexpressed in colorectal, head and neck, breast and oesophageal cancers, as well as in melanomas and lymphomas ( Supplementary Fig. 17a and Supplementary Table 8 ). Similarly, we observed an upregulation of GSTO1 mRNA in different cancer cell lines (HCT116, MDA-MB-435 and MDA-MB-231) by analysing transcript data in BioGPS ( Supplementary Fig. 17b ). To determine the significance of such overexpression, we evaluated the effect of silencing GSTO1 on cancer cell viability. Treatment with GSTO1-specific siRNA significantly decreased the viability of HCT116 cancer cells ( Fig. 3a ). These results were further replicated in different cancer cell lines ( Supplementary Fig. 18b ). HCT116 cells treated with C1-27 also showed a decrease in cell viability in a dose-dependent manner ( Fig. 3b ). Other top GSTO1 inhibitors too showed cytotoxicity in a panel of cancer cell lines ( Supplementary Table 9 ). Of note, C1-27 inhibited the clonogenic survival of HCT116 cells at sub-micromolar concentrations ( Fig. 3c ). Furthermore, at sub-cytotoxic concentrations, the size of the colonies was reduced, suggesting an effect on cell proliferation. To confirm this, we analysed the effect on cell cycle progression by flow cytometry. Treatment with 5 μM C1-27 for 24 h resulted in an increase in the S-phase population, with a concomitant decrease in the G0/G1 population ( Fig. 3d ). An activation of caspases was also detected ( Fig. 3e ). Since GSTO1 overexpression has been implicated in drug resistance, particularly to platinum compounds [7] , [18] , [19] , we tested the effects of GSTO1 inhibitors in combination with cisplatin in HCT116 cells. C1-27 was able to significantly enhance cisplatin-induced cytotoxicity in a clonogenic assay, at non-cytotoxic concentrations ( Fig. 3f ). Although siRNA studies show that GSTO1 is important for HCT116 cancer cell viability, knockdown of GSTO1 did not appear to affect C1-27 cytotoxicity, suggesting that other targets of C1-27 also may contribute to its cytotoxicity and have a compensatory effect ( Supplementary Fig. 18c ). 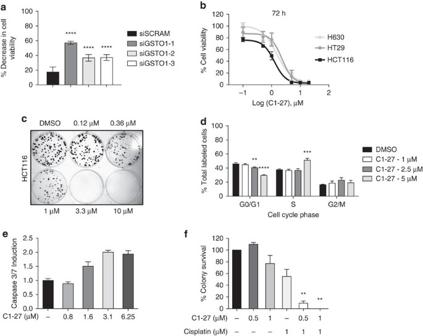Figure 3: GSTO1 inhibition impedes cancer cell viability. (a) GSTO1 knockdown decreases HCT116 cell viability. In all, 4,000 cells per well were transfected with three different GSTO1-specific siRNAs (10 nM) and cell viability was assessed by MTT assay. Data are mean of 10 replicate wells (error bars, s.e.m.). (b)C1-27inhibited cancer cell viability, as measured by MTT assay. Data are mean±s.d. of two independent experiments with duplicate wells. (c)C1-27significantly inhibited clonogenicity of HCT116 cells. Representative colony plate of three independent experiments is shown. (d) Cell cycle progression in HCT116 cells, treated with 5 μMC1-27for 24 h, was analysed by flow cytometry. Mean per cent of propidium iodide-labelled cells in each cell cycle phase calculated from three independent experiments (error bars, s.d.). (e) Induction of apoptosis by 24 hC1-27treatment, assessed by ApoTox-Glo triplex assay. Data are mean of triplicate wells (error bars, s.d.). (f)C1-27enhances cisplatin-induced cytotoxicity. HCT116 cells were treated with indicated concentrations ofC1-27and cisplatin for 24 h. Per cent colony survival from three independent colony formation assay experiments was assessed (error bars, s.d.). **P<0.01; ***P<0.001; ****P<0.0001, analysed by two-tailed, unpaired Student’st-test assuming unequal variance. Figure 3: GSTO1 inhibition impedes cancer cell viability. ( a ) GSTO1 knockdown decreases HCT116 cell viability. In all, 4,000 cells per well were transfected with three different GSTO1-specific siRNAs (10 nM) and cell viability was assessed by MTT assay. Data are mean of 10 replicate wells (error bars, s.e.m.). ( b ) C1-27 inhibited cancer cell viability, as measured by MTT assay. Data are mean±s.d. of two independent experiments with duplicate wells. ( c ) C1-27 significantly inhibited clonogenicity of HCT116 cells. Representative colony plate of three independent experiments is shown. ( d ) Cell cycle progression in HCT116 cells, treated with 5 μM C1-27 for 24 h, was analysed by flow cytometry. Mean per cent of propidium iodide-labelled cells in each cell cycle phase calculated from three independent experiments (error bars, s.d.). ( e ) Induction of apoptosis by 24 h C1-27 treatment, assessed by ApoTox-Glo triplex assay. Data are mean of triplicate wells (error bars, s.d.). ( f ) C1-27 enhances cisplatin-induced cytotoxicity. HCT116 cells were treated with indicated concentrations of C1-27 and cisplatin for 24 h. Per cent colony survival from three independent colony formation assay experiments was assessed (error bars, s.d.). ** P <0.01; *** P <0.001; **** P <0.0001, analysed by two-tailed, unpaired Student’s t -test assuming unequal variance. Full size image Gene expression signatures of C1-27 and GSTO1 knockdown To identify pathways regulated by GSTO1 and to understand the mechanism of its antiproliferative effects, we used the nascent RNA Bru-seq method [27] to profile gene expression changes that occur in response to GSTO1 knockdown and inhibition. In HCT116 cells treated with siGSTO1 for 24 h, 751 genes were upregulated and 1,108 genes were downregulated by over 1.4-fold, compared with control cells ( Fig. 4a ). CHAC1 (cation transport regulator homologue 1) was one of the most significantly upregulated genes in response to GSTO1 knockdown ( Supplementary Table 10 ). In addition, several stress- and metabolism-related genes such as oxidative stress-induced growth inhibitor 1 ( OSGIN1 ), solute carrier family 7 member 11 ( SLC7A11 ), haem oxygenase 1 ( HMOX1 ) and glucose-6-phosphate dehydrogenase ( G6PD ) were also induced. Consistent with the Bru-seq results, GSTO1 knockdown markedly induced SLC7A11 and HMOX1 protein expression at 24 h ( Fig. 4b ). Among the genes downregulated in response to GSTO1 siRNA, coagulation factor III ( F3 ), thrombospondin 1 ( THBS1 ), cysteine-rich angiogenic inducer ( CYR61 ) and bone morphogenetic protein 4 ( BMP4 ), related to blood coagulation and blood vessel morphogenesis, were markedly decreased ( Supplementary Table 11 ). Of note, transcription of cyclin-dependent kinase inhibitor, p21 ( CDNK1A ) was significantly upregulated in response to GSTO1 knockdown while that of the cell cycle regulatory proteins cyclin D1 ( CCND1 ), cyclin E1 ( CCNE1 ), as well as Myc were found downregulated (GEO accession No. GSE85899 ). 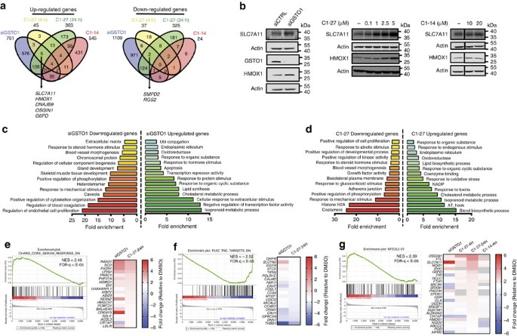Figure 4: Analysis of gene expression following C1-27 treatment and GSTO1 knockdown. (a) Venn diagram of genes upregulated (left) and downregulated (right) over 1.4-fold or more after treatment withC1-27(1 μM), the inactive analogueC1-14(10 μM) or GSTO1 knockdown (siGSTO1), as measured by Bru-seq. (b) Western blotting of SLC7A11 and HMOX1 expression after 24 h treatment of HCT116 cells with siGSTO1,C1-27orC1-14at indicated concentrations. (c,d) Pathway analysis of differentially transcribed genes following GSTO1 knockdown (c) andC1-27(24 h) treatment (d). Functional terms represented by genes downregulated (left) and upregulated (right) by at least 1.4-fold and with a count of four or more genes, as analysed using DAVID (david.abcc.ncifcrf.gov) are shown. (e) GSEA plot show enrichment of genes upregulated by siGSTO1 and 24 hC1-27treatment in the ‘CHANG_CORE_SERUM_RESPONSE_DN’30signature. (f) GSEA plot shows significant enrichment of genes downregulated by siGSTO1 andC1-27treatment in the tenascin-C-associated gene signature41. (g) GSEA plot shows enrichment of ‘NFE2L2.V2’ (ref.31) stress-response signature among genes upregulated byC1-27treatment. In each panel, nominalPvalues and false discovery rate-qvalues are indicated. Heatmaps depict the relative expression levels of top genes enriched in each gene set in siGSTO1-,C1-27-(4 or 24 h treatment) orC1-14-treated HCT116 cells as indicated. Grey cells denote genes with no transcription detected. Figure 4: Analysis of gene expression following C1-27 treatment and GSTO1 knockdown. ( a ) Venn diagram of genes upregulated (left) and downregulated (right) over 1.4-fold or more after treatment with C1-27 (1 μM), the inactive analogue C1-14 (10 μM) or GSTO1 knockdown (siGSTO1), as measured by Bru-seq. ( b ) Western blotting of SLC7A11 and HMOX1 expression after 24 h treatment of HCT116 cells with siGSTO1, C1-27 or C1-14 at indicated concentrations. ( c , d ) Pathway analysis of differentially transcribed genes following GSTO1 knockdown ( c ) and C1-27 (24 h) treatment ( d ). Functional terms represented by genes downregulated (left) and upregulated (right) by at least 1.4-fold and with a count of four or more genes, as analysed using DAVID ( david.abcc.ncifcrf.gov ) are shown. ( e ) GSEA plot show enrichment of genes upregulated by siGSTO1 and 24 h C1-27 treatment in the ‘CHANG_CORE_SERUM_RESPONSE_DN’ [30] signature. ( f ) GSEA plot shows significant enrichment of genes downregulated by siGSTO1 and C1-27 treatment in the tenascin-C-associated gene signature [41] . ( g ) GSEA plot shows enrichment of ‘NFE2L2.V2’ (ref. 31 ) stress-response signature among genes upregulated by C1-27 treatment. In each panel, nominal P values and false discovery rate- q values are indicated. Heatmaps depict the relative expression levels of top genes enriched in each gene set in siGSTO1-, C1-27- (4 or 24 h treatment) or C1-14 -treated HCT116 cells as indicated. Grey cells denote genes with no transcription detected. Full size image To explore the biological functions of these genes, we performed functional enrichment analysis using database for annotation, visualization and integrated discovery (DAVID) [28] . Genes that were upregulated by more than 1.4-fold in response to GSTO1 knockdown showed an enrichment of pathway terms related to lipid synthesis, sterol metabolism and transcriptional repression. In addition, pathways related to hormone stimulus, oxidative stress and endoplasmic reticulum were also enriched ( Fig. 4c ). Among the genes downregulated by more than 1.4-fold, a significant enrichment of functional pathways related to caveola, cytoskeleton organization, blood vessel and coagulation, as well as chromosomal proteins was observed. To further delineate pathways that are responsive to GSTO1 knockdown, we performed gene set enrichment analysis (GSEA) using the Bru-seq data ( Supplementary Tables 12 and 13 ). Genes upregulated by GSTO1 siRNA showed significant enrichment of amino-acid deprivation response-related gene sets [29] . A wound-healing-related gene set, described by Chang et al . [30] , representing genes negatively regulated in the fibroblast core serum response, was also strongly enriched among the genes upregulated by GSTO1 knockdown ( Fig. 4e ). Genes downregulated by siGSTO1 showed an enrichment of gene sets relating to tenascin-C signalling and oestrogen response ( Fig. 4f ). We also examined gene expression changes induced by C1-27 in HCT116 cells after 4 and 24 h treatment to observe the early and late response to GSTO1 inhibition, respectively ( Supplementary Tables 14–17 and 20–23 ). By comparing these transcriptional changes with those induced by an inactive analogue, C1-14 ( Supplementary Fig. 19 and Supplementary Tables 18, 19 and 24 ), we further sought to discriminate between the on-target and off-target effects of C1-27 . The early effects of GSTO1 inhibition by C1-27 (4 h treatment) predominantly involved induction of several stress-response-associated genes ( OSGIN1 , HMOX1 , SLC7A11 , DNAJB9 and so on) ( Supplementary Table 14 ). GSEA analysis revealed a significant enrichment of a NRF2 stress-response signature [31] . Sustained GSTO1 inhibition for 24 h also resulted in a similar stress-response signature ( Fig. 4g and Supplementary Table 16 ). Western blotting further showed that C1-27 markedly increased SLC7A11 and HMOX1 expression, while the inactive control had no effect ( Fig. 4b ). More importantly, 24 h treatment of HCT116 cells with C1-27 resulted in transcriptional changes that were more similar to those observed with GSTO1 knockdown ( Fig. 4a ), with <12% overlap with the inactive control, C1-14 . A comparison of C1-27 -treated (24 h) and GSTO1 siRNA-treated transcriptomes showed an overlap of 111 commonly upregulated genes and 126 commonly downregulated genes with more than 1.4-fold change in expression. GSEA of genes upregulated by 24 h treatment with C1-27 likewise showed a significant enrichment of the wound-healing gene set ( Fig. 4e and Supplementary Table 22 ). Genes downregulated after 24 h treatment with C1-27 also showed significant enrichment of the tenascin-C signalling gene set ( Fig. 4f and Supplementary Table 23 ). Pathway analysis of the upregulated and downregulated genes using DAVID showed an enrichment of functional terms related to cholesterol metabolism, NADP, response to oxidative stress and response to mechanical stimulus, adherens junction and blood vessel morphogenesis, respectively ( Fig. 4d ). C1-27 suppresses human colon cancer xenograft growth in vivo To test whether C1-27 had in vivo efficacy, we initially evaluated its effects in a human colon cancer cell line xenograft model. C1-27 (20–45 mg kg −1 ) was administered as a single agent to nude mice bearing HCT116 xenografts. After 5 weeks of treatment, tumour growth was significantly inhibited in C1-27 -treated mice compared with the vehicle-treated group ( P <0.05) ( Fig. 5a ). C1-27 treatment was generally well tolerated by mice up to 45 mg kg −1 , with no overt signs of toxicity and no significant variations in average body weights throughout the duration of the study ( Fig. 5b ). Haematoxylin and eosin staining of the tumour sections from C1-27 -treated mice showed extensive regions of necrosis compared with control ( Fig. 5c ). To further assess any treatment-related toxicity, kidney and liver tissue sections from control and C1-27 -treated mice were examined by histology. Haematoxylin and eosin staining showed no gross morphological differences ( Fig. 5d ). We further evaluated the antitumour efficacy of C1-27 in a more clinically relevant colorectal cancer patient-derived xenograft (PDX) model. The KRAS-mutant CRM-13-180 PDX model, which showed a high GSTO1 expression, was chosen for the study ( Supplementary Fig. 20a ). C1-27 showed potent and selective inhibition of GSTO1 in these cells ( Supplementary Fig. 20b ). In vivo , C1-27 resulted in a relatively modest but statistically significant inhibition of tumour growth (per cent treated/control (% T / C )=67), which was comparable to the tumour growth inhibition shown by oxaliplatin (L-OHP; % T / C =63) ( Fig. 5e ). On the other hand, arsenic trioxide (As 2 O 3 ) and SC-144 showed significant tumour growth reduction (% T / C =29 and 32, respectively) and tumour growth delay ( T − C >10 days). The maximum C1-27 treatment-related weight loss during the course of the study did not exceed 12% ( Supplementary Fig. 20c ). We further examined in vivo binding of C1-27 to GSTO1 using the PDX tumour tissue homogenates. BODIPY- C1-27A labelling of GSTO1 was decreased in C1-27 -treated tumours compared with the control group ( Fig. 5f ). Furthermore, expression of SLC7A11, a GSTO1 and C1-27 target gene, was increased in C1-27 -treated tumours indicating target engagement ( Fig. 5g ). Taken together, these results demonstrate that C1-27 targets GSTO1 in tumours and shows promising antitumour activity in both cell line xenograft and PDX models of colorectal cancer, without gross systemic toxicities. 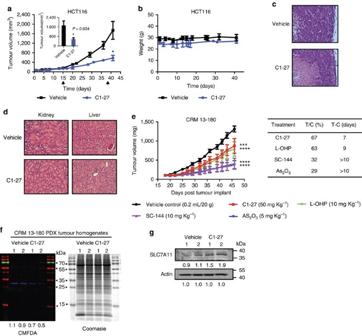Figure 5: C1-27 inhibits colorectal cancer tumour growthin vivo. (a) Tumour growth curves of HCT116 tumour-bearing nude mice treated with vehicle (n=5) orC1-27(n=3). Data shown are mean tumour volumes (error bars, s.e.m.). Arrows indicate dose escalation (treatment schedule is described in the Methods section). Significant reduction in tumour volumes was observed on day 41 ofC1-27treatment (*P<0.05, analysed by one-way analysis of variance (ANOVA)). (b) Mean body weights ofC1-27-and vehicle-treated HCT116 tumour-bearing mice over the duration of treatment (error bars, s.e.m.). (c)C1-27-treated tumours showed extensive areas of necrosis, as seen by haematoxylin/eosin staining of tumour sections fromC1-27-and vehicle-treated mice. Representative image of four independent sections is shown. (d) Haematoxylin/eosin staining of liver and kidney sections showed no gross signs of systemic toxicity. (e) Comparison of tumour growth curves in colorectal cancer PDX model CRM 13–180. NCR nude mice implanted with CRM 13–180 tumour fragments were treated withC1-27, SC-144, As2O3or vehicle (n=5/group), on a 5 days on/2 days off schedule by intraperitoneal injection. L-OHP (n=5) was administered once a week. Data shown are mean tumour volumes (error bars, s.e.m.; ***P=0.0011; ****P<0.0001, analysed by two-way ANOVA). Table shows comparison of efficacies of treatments.T/C(%) represents the relative size of the median tumour burden of the treated (T) versus vehicle control (C) groups on the last day of treatment.T−C represents the difference in days for the treated (T) and vehicle control (C) tumour burden to reach a median size of 750 mg. (f) Fluorescence scan of BODIPY-C1-27Abinding in CRM 13–180 tumour homogenates from vehicle andC1-27-treated mice. Normalized relative GSTO1 band intensities shown below. (right) Coomasie staining of the gel. (g) Western blotting of SLC7A11 expression in CRM 13–180 tumour homogenates from vehicle andC1-27-treated mice. Normalized relative densities computed using ImageJ are shown below. Figure 5: C1-27 inhibits colorectal cancer tumour growth in vivo . ( a ) Tumour growth curves of HCT116 tumour-bearing nude mice treated with vehicle ( n =5) or C1-27 ( n =3). Data shown are mean tumour volumes (error bars, s.e.m.). Arrows indicate dose escalation (treatment schedule is described in the Methods section). Significant reduction in tumour volumes was observed on day 41 of C1-27 treatment (* P <0.05, analysed by one-way analysis of variance (ANOVA)). ( b ) Mean body weights of C1-27- and vehicle-treated HCT116 tumour-bearing mice over the duration of treatment (error bars, s.e.m.). ( c ) C1-27 -treated tumours showed extensive areas of necrosis, as seen by haematoxylin/eosin staining of tumour sections from C1-27- and vehicle-treated mice. Representative image of four independent sections is shown. ( d ) Haematoxylin/eosin staining of liver and kidney sections showed no gross signs of systemic toxicity. ( e ) Comparison of tumour growth curves in colorectal cancer PDX model CRM 13–180. NCR nude mice implanted with CRM 13–180 tumour fragments were treated with C1-27 , SC-144, As 2 O 3 or vehicle ( n =5/group), on a 5 days on/2 days off schedule by intraperitoneal injection. L-OHP ( n =5) was administered once a week. Data shown are mean tumour volumes (error bars, s.e.m. ; *** P =0.0011; **** P <0.0001, analysed by two-way ANOVA). Table shows comparison of efficacies of treatments. T / C (%) represents the relative size of the median tumour burden of the treated ( T ) versus vehicle control ( C ) groups on the last day of treatment. T −C represents the difference in days for the treated ( T ) and vehicle control ( C ) tumour burden to reach a median size of 750 mg. ( f ) Fluorescence scan of BODIPY- C1-27A binding in CRM 13–180 tumour homogenates from vehicle and C1-27 -treated mice. Normalized relative GSTO1 band intensities shown below. (right) Coomasie staining of the gel. ( g ) Western blotting of SLC7A11 expression in CRM 13–180 tumour homogenates from vehicle and C1-27 -treated mice. Normalized relative densities computed using ImageJ are shown below. Full size image Through extensive small-molecule screening, biochemical assays and X-ray crystallography, we have identified several potent GSTO1 inhibitors. Co-crystal structures of GSTO1 bound to inhibitors showed a covalent association with the active site cysteine (C32) with additional hydrophilic and hydrophobic interactions in the H-site. Although reactive electrophiles such as chloroacetamides are generally considered to be promiscuous in target binding, we demonstrated here using a BODIPY-labelled analogue that the chloroacetamide-based GSTO1 inhibitor C1-27 exhibited a low degree of nonspecific reactivity. In addition to GSTO1, C1-27 showed binding also to PDI. However, binding and enzyme inhibition studies revealed a 100-fold more potent affinity for GSTO1 than PDI. A previous study also reported a similar low random reactivity of selected reactive electrophiles [32] . Although not characterized in this study, we expect these inhibitors to also bind GSTO2, since it shares 64% sequence identity with GSTO1. In vitro mechanistic studies also showed that the lead compound C1-27 acts as a slow-turnover substrate, though the significance of this mechanism is currently unclear. GSTO1 overexpression has been previously reported in several cancers, as well as in drug-resistant cell lines [7] , [16] , [17] , [18] , [19] . We show here in a panel of cancer cell lines that GSTO1 knockdown reduced cancer cell viability. RNA expression profiling also showed a significant increase in CDKN1A (p21), a p53 target gene coding for a cell cycle inhibitor, together with a decrease in the transcription of CCND1 , CCNE1 and Myc . In accordance with this, pathway analysis of the RNA transcriptome identified oestrogen-mediated S-phase entry, p53 signalling and G1/S checkpoint regulation as canonical pathways significantly modulated in response to GSTO1 knockdown ( Supplementary Fig. 21 ). Interestingly, the pro-survival function of GSTO1 in cancer cells appeared to be cancer- or cell type-specific. We observed that KRAS mutant cancer cell lines (HCT116 and H460) and MDA-MB-435, with a high GSTO1 expression, were sensitive to GSTO1 knockdown, but not MCF7 cells ( Supplementary Fig. 18 ). Similarly, T47D cells have also previously been reported to be devoid of mature GSTO1 (ref. 33 ), with no effect on cell viability. We further observed that the lead GSTO1 inhibitor C1-27 blocked cancer cell proliferation, caused cytotoxicity, inhibited cell cycle progression and increased the sensitivity of cancer cells to cisplatin. KRAS mutant cancer cell lines (HCT116 and Panc-1) were more sensitive to GSTO1 inhibition ( Supplementary Table 25 ). Furthermore, the cell death induced by C1-27 appeared to be Ras-signalling-dependent ( Supplementary Fig. 22 ). It is of interest to note that a class of tertiary α-chloroacetamide-containing compounds such as RSL3 has previously been shown to induce a unique iron-dependent, oxidative, non-apoptotic cell death, selectively in KRAS-mutant cells, through covalently inhibiting glutathione peroxidase 4 (refs 34 , 35 , 36 ). Finally, C1-27 showed in vivo efficacy in both HCT116 cell line xenograft and PDX models of colorectal cancer. We also noted that GSTO1 expression was higher in several colorectal cancer patient tumours as compared with normal colon tissue, consistent with our bioinformatics analysis ( Supplementary Fig. 20a ). GSTO1 has been shown to play a significant role in the protein glutathionylation cycle exhibiting both glutathionylation and deglutathionylation activities [11] , [15] . Mitochondrial F 0 /F 1 ATPase β subunit has been shown to be glutathionylated by GSTO1 (ref. 9 ), while β-actin has been reported to be specifically deglutathionylated by it [11] . Similarly, silencing GSTO1 or inhibition of its catalytic activity increased cellular levels of protein glutathionylation [14] . On the other hand, GSTO1 also catalysed rapid glutathionylation of cellular proteins during oxidative stress [11] , [15] . Interestingly, GSTO1 was identified as one of the potential cellular targets of piperlongumine, an electrophilic compound exerting selective cytotoxicity against cancer cells through an oxidative cell death mechanism ( Supplementary Table 25 ) [37] . Piperlongumine and its analogues have also been shown to increase the levels of protein glutathionylation [38] . Together, these findings suggest a role for GSTO1 in regulating cell signalling and redox homeostasis through affecting the S -glutathionylation status on its target proteins. While a role in cellular stress response is emerging, the cellular targets of GSTO1 and its functions have not been fully understood. To address this, we performed transcription profiling using Bru-seq and identified genes involved in cellular stress response, steroid metabolism, transcription and cytoskeleton organization as significantly altered by both GSTO1 siRNA and C1-27 . Our data suggest that GSTO1 depletion results in cellular stress with a significant increase in the expression of various NRF2 target genes such as OSGIN1 , SLC7A11 and HMOX1 . We further confirmed their expression by western blotting, thus validating the nascent RNA-profiling results. A previous study in macrophage cells also similarly showed that GSTO1 knockdown as well as GSTO1 inhibitor M175 (ref. 21 ) induced antioxidant genes after stimulation with lipopolysachcharide [14] . In particular, our nascent transcriptome analyses showed a significant increase in SLC7A11 gene transcription in both C1-27 - and GSTO1 siRNA-treated cells. SLC7A11 encodes xCT, a cationic amino-acid transporter that is part of the cysteine- and glutamate-specific cationic antiporter, system X c − . Its transcription is regulated by NRF2 and system X c − inhibition. We also observed a 23-fold increase in CHAC1 transcription with GSTO1 knockdown but not with C1-27 treatment. CHAC1 functions as a γ-glutamylcyclotransferase catalysing glutathione degradation [39] . It is also induced during endoplasmic reticulum stress, regulated by the ATF4-CHOP branch of the unfolded protein response, and elicits an apoptotic response [40] . Since GSTO1 knockdown has been known to result in increased protein glutathionylation [14] , glutathione depletion by CHAC1 could possibly contribute in restoring the glutathionylation balance. Pathway analysis further identified cholesterol metabolism ( INSIG1 , FDFT1 , SREBF1 , LDLR and so on) as being modulated by both C1-27 and GSTO1 knockdown. Interestingly, many of these genes involved in cholesterol homeostasis were also implicated in a gene signature related to the fibroblast core serum response [30] . GSTO1 knockdown as well as the small-molecule GSTO1 inhibitor C1-27 also caused downregulation of the Wnt inhibitor Dickkopf 1 ( DKK1 ), thombospondin 1 ( THBS1 ), the cysteine-rich angiogenic inducer CYR61 and caveolae scaffolding proteins CAV1 and CAV2 , among others. GSEA analysis further revealed significant enrichment of a tenascin-C-induced gene signature. Tenascin-C is an extracellular matrix glycoprotein that modulates cell adhesion and migration [41] . Since GSTO1 has been known to cause de-glutathionylation of β-actin impeding its polymerization into filamentous actin [11] , such a downregulation of molecules involved in cytoskeleton organization and adhesion is particularly interesting. Of note, GSTO1 was identified as one of the cellular targets of locostatin, an oxazolidinone-based cell migration inhibitor, although its role in cell migration has not been well characterized [42] . While the mechanism by which GSTO1 interacts with these genes and pathways remains to be fully characterized, GSTO1 catalytic activity appears to be important for this regulation. In addition to these cellular functions, GSTO1 has been shown to play a significant role in the regulation of IL-1β processing and secretion [12] , [13] . While the exact mechanism is not fully understood, GSTO1 appears to be associated with the early responses in the pro-inflammatory pathway, influencing oxidative and metabolic changes [43] . Although beyond the scope of discussion in this paper, we found that C1-27 and several of the potent GSTO1 inhibitors inhibited the secretion of mature IL-1β from activated monocytic cells ( Supplementary Fig. 23 ). We further observed that pretreatment with C1-27 inhibited the transcriptional induction of pro-IL-1β in response to inflammatory stimulus such as the bacterial endotoxin, lipopolysachcharide. These findings further extend the utility of GSTO1 inhibitors as anti-inflammatory agents. Inhibition of IL-1β secretion by GSTO1 inhibitors also has exciting implications on tumour progression and tumour-immune cell crosstalk in the microenvironment. In conclusion, we have shown that GSTO1 is a novel and exciting target for developing anticancer and anti-inflammatory agents. Our nascent RNA expression studies suggest, for the first time, novel roles for GSTO1 in cell signalling. GSTO1 inhibitors show efficacy against cancer cells in both in vitro and in vivo models and enhance the cytotoxic effects of cisplatin. Moreover, our potent inhibitors serve as valuable tools to investigate the role of GSTO1 in cancer and other pathologies, as well as to uncover additional functions in the cell. Further studies are in progress to design clinically viable candidates through structure-based drug design approaches using the co-crystal structures of our lead inhibitors. Compounds for high-throughput screening For the similarity search and expanded screening, a diverse library of small-molecule compounds ( ∼ 1,000,000) from Asinex, Enamine and in-house collection was used. Compounds from commercial sources were purchased with a minimum purity of 90% and were stored as 50 mM stock in dimethylsulfoxide (DMSO) at −80 °C. The lead compound C1-27 was procured from Enamine (97% purity) and further characterized using mass spectrometry (electrospray ionisation mass spectrometry ( m / z ): [M] + calcd. for C 10 H 12 Cl 2 N 2 O 3 S, 309.99; found, 309.16). Substrate for GSTO1 enzymatic assay, 4-NPG was synthesized as previously described [17] . Product purity was confirmed by mass spectrometry (electrospray ionisation mass spectrometry ( m / z ): [M] + calcd. for C 18 H 23 N 4 O 9 S, 471.12; found, 471.04) and Ellman’s reagent (unreacted residual glutathione <1%). Synthesis and characterization of compounds used in pilot screening and target validation are detailed in Supplementary Methods . Cell lines Colon cancer cell line HCT116 was generously provided by Dr Bert Vogelstein, Johns Hopkins Medical Institutions, Baltimore, MD. Pancreatic cancer cell line Panc-1 was obtained from Dr Alan Epstein, University of Southern California. All other cell lines were purchased from the American Type Culture Collection (Manassas, VA). MDA-MB-435 cell line was used in the GSTO1 knockdown experiment as it had high GSTO1 expression ( Supplementary Fig. 17 ). We also tested active compounds in NCI-ADR/Res cell line since GSTO1 is implicated in drug resistance. Cell lines were cultured in RPMI 1640 or Dulbecco’s minimal essential media supplemented with 10% fetal bovine serum at 37 °C in a humidified atmosphere of 5% CO 2 . All cell lines were maintained in culture under 30 passages and tested regularly for Mycoplasma contamination using PlasmoTest (InvivoGen, San Diego, CA, USA). Reagents The following reagents were purchased from Cell Signaling Technology: MEK inhibitor (PD98059); PI3K inhibitor (LY294002); and JNK inhibitor (SP600125). Cisplatin was purchased from Sigma. CellTracker Green (CMFDA) was purchased from Invitrogen (Thermo Fisher Scientific). Erastin and Piperlongumine were purchased from Sigma and LKT labs, respectively. L-OHP and As 2 O 3 were purchased from BioTang Inc. SC-144 is a GP130 inhibitor previously identified by our lab [44] . Catalogue numbers and dilutions of antibodies used in this study are summarized in Supplementary Table 26 . Drugs and formulations for in vivo experiments C1-27 and SC-144 were dissolved in DMSO to make a stock solution. Aliquots of the stock solutions were stored at −20 °C. On each day of treatment, an aliquot of each compound was thawed and diluted using propylene glycol (60% total volume) and 0.9% normal saline (30% total volume). In the HCT116 xenograft study, C1-27 was diluted using peanut oil. Arsenic trioxide (As 2 O 3 ) was dissolved in 1 N NaOH to make a 50 mg ml −1 stock solution and stored at 4 °C. On each day of treatment, the As 2 O 3 stock solution was diluted in saline and the pH adjusted using 1 N HCl. L-OHP was stored at −20 °C as a powder and was dissolved in 5% glucose on each day of treatment. Bioinformatics analysis GSTO1 gene expression in normal and cancer tissues was analysed using Oncomine cancer microarray database ( www.oncomine.org ) across various cancer subtypes using a cancer versus normal differential analysis. Within the same cancer subtype, meta-analysis was done to compare different studies and assess overall significance of GSTO1 expression. Data sets used in the study are summarized in Supplementary Table 8 . Cancer subtypes with more than one study, P <0.05 and fold change >1.5 were used as inclusion criteria for further analysis. For correlation analysis, normalized median-centred values for GSTO1 and IL-1β expression in each microarray study was plotted and Pearson’s correlation coefficient was computed using Prism 6.0. GSTO1 mRNA expression in different cancer cell lines was assessed using BioGPS ( www.biogps.org ). siRNA experiments GSTO1 siRNA (Trilencer-27) and scrambled control siRNA were purchased from Origene (Rockville, MD). Cells were transfected with GSTO1 siRNA (siGSTO1-1, siGSTO1-2 and siGSTO1-3) or scrambled control siRNA (siSCRAM) using Lipofectamine RNAiMAX (Invitrogen, Thermo Fisher Scientific) following the manufacturer’s instructions. GSTO1 knockdown in HCT116 cells was confirmed by in-gel fluorescence using CMFDA (500 nM) 48 and 72 h post transfection. Effect on cell viability was assessed 72 h after transfection with GSTO1 siRNA or siSCRAM by 3-(4,5-dimethylthiazol-2-yl)-2,5-diphenyltetrazolium bromide (MTT) assay and normalized to mock-transfected control (transfection reagent). Expression and purification of GSTO1 for screening Human GSTO1-1 plasmid was a kind gift from Dr Philip Board, John Curtin School of Medical Research, Australian National University. Recombinant GSTO1-1 was expressed in Escherichia coli M15 (Rep4) cells (Qiagen) and purified as described previously [5] , [45] . Briefly, GSTO1-1 pQE30 plasmid was transformed into M15 cells, which were grown in Luria-Bertani broth supplemented with 100 μg ml −1 ampicillin and 25 μg ml −1 kanamycin at 37 °C to an OD 600 of ∼ 0.8 and induced with 0.1 mM isopropyl thio- β - D -galactoside for 4 h. Bacterial cells were collected by centrifugation at 4,000 g for 20 min at 4 °C and the cell pellet was resuspended in buffer (50 mM NaH 2 PO 4 and 300 mM NaCl, pH 6.0). Cells were lysed by sonication and the cleared supernatant was purified using Ni-NTA resin. The purified enzyme was dialysed against 20 mM Tris-HCl and 60 mM NaCl, pH 8.0. Protein purity was assessed by SDS–PAGE. Expression and purification of GSTO1 for crystallization For crystallization, GSTO1 residues 1–241 were cloned into an expression construct containing an N-terminal 6xHis tag followed by a tobacco etch virus (TEV) protease cleavage site and expressed in E. coli Rosetta 2(DE3) cells. The cells were lysed in 25 mM Tris-HCl (pH 7.5), 200 mM NaCl, 0.1% β-mercaptoethanol, 10 mM MgCl 2 , 2.1 mM leupeptin, 1.53 mM aprotinin and 50 U of benzonase (Novagen). Cleared lysate was incubated with Ni-NTA resin (Qiagen) at 4 °C for 1 h. The column was washed with 25 mM Tris (pH 7.5), 200 mM NaCl and 10 mM imidazole, and eluted with 25 mM Tris (pH 7.5), 200 mM NaCl and 500 mM imidazole. Eluate incubated with TEV protease was dialysed against 25 mM Tris (pH 7.5), 150 mM NaCl and 1 mM DTT overnight at 4 °C, then incubated with Ni-NTA resin for 1 h to remove the His-tagged protease. The Ni-NTA flow-through was concentrated and applied to a Superdex 200 column equilibrated with 25 mM Tris 7.5, 60 mM NaCl and 5 mM DTT. The purified protein was concentrated to 2 mg ml −1 and stored at −80 °C. Crystallization and structure determination Before crystallization, GSTO1 was dialysed against 25 mM Tris 7.5, 60 mM NaCl and 1 mM DTT. The GSTO1– C1-27 complex was created by incubating GSTO1 (27 mg ml −1 ) in a 1:1.5 molar ratio with C1-27 at 4 °C for 48 h. The complex crystallized under sitting drop vapour diffusion against 24% PEG 3350 and 100 mM MES (pH 6.5) with a drop configuration of 2 μl of complex, 1.8 μl well and 0.2 μl 40% tert-butanol. The GSTO1– C1-31 complex was formed by incubating GSTO1 (2.66 mg ml −1 ) in a 1:1.5 molar ratio with C1-31 at 4 °C for 24 h, then concentrated to 23.9 mg ml −1 before crystallization. Crystals formed from drops containing equal volumes of complex and well solution (22.5% PEG 3350, 90 mM MES (pH 6.5) and 4% tert-butanol). For the GSTO1– C4-10 complex, GSTO1 (2.66 mg ml −1 ) was incubated in a 1:1.5 molar ratio with C4-10 for 24 h at 4 °C then concentrated to 26.2 mg ml −1 . Crystals of the complex grew from sitting drops containing equal volumes of protein complex and well solution (22.5% PEG 3350, 90 mM MES (pH 6.5) and 10 mM BaCl 2 ). All crystals grew at 20 °C. The GSTO1– C1-27 and GSTO1– C1-31 crystals were cryoprotected with 30% PEG and 100 mM MES (pH 6.5) before data collection; GSTO1– C4-10 crystals had no additional cryoprotection. Diffraction data for GSTO1– C1-27 , GSTO1– C1-31 and GSTO1– C4-10 were collected on LS-CAT lines (21-ID-D and 21-ID-G) at the Advanced Photon Source at Argonne National Laboratory and processed with HKL2000 (ref. 46 ). The structures were solved by molecular replacement (MOLREP [47] ) using GSTO1 (PDB ID: 1EEM) as a search model. Three monomers of GSTO1 were present in the asymmetric unit of the GSTO1– C1-27 and GSTO1– C4-10 crystals, while a dimer was present in the GSTO1– C1-31 crystal. Iterative rounds of electron density fitting and refinement were completed using Coot [48] and Buster [49] , respectively. Difference electron density maps contoured to 3 σ showed the presence of inhibitor molecules covalently bound to C32 in all protein chains. The coordinates and geometric restraints for each inhibitor were created from smiles using Grade [49] with the qm+mogul option. Statistics for the refined structures are given in Supplementary Table 27 . Residues 1–4 were disordered in all structures along with loop residues 133–135 in C1-31 . The structures were validated using Whatcheck [50] , Molprobity [51] and Pavarti [52] . GSTO1 enzyme activity assay Enzyme activity was measured by monitoring the reduction of 4-NPG to 4-nitroacetophenone by GSTO1. Briefly, in a 200 μl reaction volume, 5 μg ml −1 recombinant GSTO1 in reaction buffer (100 mM Tris (pH 8.0), 1.5 mM EDTA and 1 mM DTT) was incubated with DMSO or different concentrations of inhibitors for 30 min at 37 °C. A volume of 4-NPG (final concentration of 1 mM) was added to the reaction and decrease in absorbance at 305 nm was recorded on an Envision multilabel plate reader (Perkin Elmer). In-gel fluorescence binding assay Primary screening of GSTO inhibitors was based on competitive inhibition of CMFDA binding to endogenous GSTO. Briefly, HCT116 p53+/+ cells (4 × 10 4 per well) were coated in a 12-well plate. After overnight attachment, cells were treated with test compounds at 10 μM for 2 h at 37 °C followed by addition of 500 nM CMFDA for 1 h. Cells were then washed with PBS and lysed using Cell Lytic M buffer (Sigma). A unit of 15 μg of whole-cell protein extracted was boiled with Laemmli sample buffer and resolved on a 15% polyacrylamide gel. Gels were immediately scanned on a Typhoon variable mode imager (Amersham Bioscience). Quantification of fluorescent band intensity was done using Image Quant 5.2 software. Compounds that showed at least 50% inhibition of CMFDA binding to GSTO were selected for dose–response determinations. Similarly, in vitro binding assay with recombinant GSTO1 was performed using 1 μM GSTO1 in reaction buffer (100 mM Tris (pH 8.0), 1.5 mM EDTA and 1 μM DTT) incubated with compounds for 30 min at 37 °C and with CMFDA (500 nM) for an additional 30 min. For selectivity studies, recombinant GSTO1 (1 μM), PDI (1 μM), BSA (1 μM) or GRP78 (1 μM) in reaction buffer were incubated with C1-27 or DMSO for 30 min at 37 °C, followed by incubation with CMFDA (500 nM), BODIPY- C1-27A (1 μM) or DMSO for 30 min. Similarly, CRM 13–180 PDX tumour tissue from mice treated with vehicle or C1-27 was homogenized in Cell lytic M buffer and 20 μg of protein was incubated with CMFDA (500 nM) for 1 h. The reactions were quenched by boiling with Laemmli sample buffer for 5 min. The samples were resolved on a 10–15% polyacrylamide gel and scanned on a Typhoon variable mode imager or on a FluorChem M System (ProteinSimple, San Jose, CA, USA). Uncropped images of key gels are presented in Supplementary Fig. 24 . Pre-incubation and dilution assay GSTO1 (2 μg) was incubated with inhibitor at a concentration of 10 × IC 50 in a 10 μl reaction volume for 30 min at 37 °C. An aliquot of 5 μl of this reaction was diluted to 180 μl with reaction buffer (100 mM Tris (pH 8.0), 1.5 mM EDTA, 1 mM DTT) to attain final concentrations of 5 μg ml −1 GSTO1 and 0.25 × IC 50 of inhibitor. 4-NPG (20 μl, 0.5 mM) was added and decrease in absorbance was monitored. % Recovery of enzyme activity was determined using a DMSO control. Duration of inhibition Receptor occupancy and duration of inhibition experiment was performed based on a previously reported method [53] . HCT116 cells were treated with C1-27 (100 nM) for 2 h, followed by drug washout. At indicated times after washout, CMFDA (500 nM) was added for 1 h and the cells were lysed and processed for in-gel fluorescence binding assay, to assess recovery of CMFDA binding to GSTO1. PDI activity assay Recombinant PDI was purified and PDI-catalysed reduction of insulin was measured as described previously [54] . Briefly, recombinant PDI protein (0.4 μM) was incubated with indicated compounds at 37 °C for 1 h in sodium phosphate buffer (100 mM sodium phosphate, 2 mM EDTA and 8 μM DTT, pH 7.0). Then the reaction mixture consisting of DTT (500 μM) and bovine insulin (130 μM) was added to the incubated PDI protein. The reduction reaction was catalysed by PDI at room temperature, and the resulting aggregation of reduced insulin B chains was measured at 620 nm. % PDI activity was calculated from absorbance values at T =0 and 80 min. Thermal-shift assay Thermal-shift assay was performed as described previously [55] . Briefly, recombinant GSTO1 was diluted into 50 mM Tris-HCl (pH 8.0) buffer containing the fluorophore 1,8 ANS (0.3 mM) to a final concentration of 0.3 mg ml −1 . A volume of 5 μl of the protein-dye mixture was dispensed into a 384-well microplate (Thermo Scientific, AB1384K), followed by addition of 5 μl of C1-27 and 3 μl of silicone oil (to avoid evaporation). Similarly, recombinant PDI was diluted to 0.3 mg ml −1 in 100 mM sodium phosphate buffer (pH 7.0) containing 0.3 mM 1,8 ANS and thermal-shift assay was performed as described above. A volume of 5 μl of 1.5% v/v DMSO and 2% v/v DMSO in respective buffers for GSTO1 and PDI were used as DMSO controls. Fluorescence intensity as a function of temperature was measured on a Thermofluor analyser (Johnson & Johnson, New Brunswick, NJ). The reaction plate was heated from 25 to 90 °C with a 1 °C min −1 increment. Triplicate measurements were made and the s.d. was within limit. Cellular thermal-shift assay Cellular thermal-shift assay was performed as described previously [56] . Briefly, HCT116 p53+/+ cells were collected, washed with PBS and diluted with cell lysis buffer (25 mM Tris-HCl (pH 7.5) and 10 mM MgCl 2 ) supplemented with complete protease inhibitor cocktail. The cell suspension was frozen and thawed three times in liquid nitrogen. The soluble fraction was separated from debris by spinning down at 20,000 g for 20 min. Cell lysate was then diluted with lysate buffer and divided into two aliquots—one treated with C1-27 (100 μM) and the other treated with 1% DMSO. After 30 min incubation at room temperature, the treated lysates were further divided into smaller aliquots (50 μl), which were then heated at different temperatures for 3 min on a Veriti thermal cycler (Applied Biosystems) followed by cooling for 3 min to room temperature. The heated lysates were centrifuged at 20,000 g for 20 min at 4°C to separate the soluble fractions from precipitates. Supernatants were quantified and analysed by western blotting. Cell viability assays Cell proliferation was assessed by a MTT assay. Cancer cells were seeded in 96-well microtitre plates and, after overnight attachment, treated with GSTO1 inhibitors. After 72 h, MTT solution (3 mg ml −1 ; 20 μl) was added to each well and cells were incubated for 3 h at 37 °C. After incubation, media from each well was removed and the dark blue formazan crystals formed by live cells were dissolved in DMSO (150 μl per well). The absorbance intensity was measured at 570 nm on a microplate reader (Molecular Devices, Sunnyvale, CA, USA). Cell viability after 24 h treatment was assessed using ApoTox-Glo triplex assay (Promega) according to the manufacturer’s protocol. At least three independent dose–response experiments with each concentration tested in triplicate were performed for each cell line. Clonogenic survival assay HCT116 cells were seeded at a density of 200 cells per well in a 6-well microtitre plate. After overnight attachment, cells were treated with different concentrations of GSTO1 inhibitors for 24 h. Colonies were allowed to grow in drug-free medium for 7 days and stained with 0.5% crystal violet. For drug combination studies, HCT116 cells (200 per well) were plated in a 12-well plate. C1-27 , cisplatin (1 μM, dissolved in 0.9% NaCl), PD98059 (10 μM), LY294002 (10 μM), SP600125 (1 μM) or desferoxamine mesylate (10 μM) were added alone or in combination and colonies were allowed to grow for 7–10 days. Cell cycle analysis Cells were seeded at a density of 0.5 × 10 6 per well in a six-well plate. After overnight attachment, cells were treated with C1-27 (5 μM) for 24 h and collected using trypsin. Cells were then washed twice with PBS containing 10% serum and fixed with 70% ethanol overnight at −20 °C. Fixed cells were washed twice in PBS containing 10% serum and stained with 50 μg ml −1 propidium iodide solution containing 100 μg ml −1 RNase A for 1 h at 37 °C. Cell cycle was analysed on a BD LSR II flow cytometer (BD Biosciences) and data were analysed using ModFit software. Caspase 3/7 assay HCT116 cells were treated with indicated concentrations of C1-27 for 24 h. Caspase activation was measured using ApoTox-Glo triplex assay reagent according to the manufacturer’s recommendation. Western blotting HCT116 cells were seeded in a six-well plate and treated with GSTO1 inhibitors for 24 h. Cells were washed with ice-cold PBS and lysed with a triple detergent lysis buffer supplemented with protease and phosphatase inhibitor cocktail. Lysate was sonicated and centrifuged at 12,000 r.p.m. for 10 min at 4 °C to remove cell debris. Total protein concentration in the supernatant was measured using BCA protein assay kit (Pierce Biotechnology). For IL-1β experiments, THP-1 cells (1 × 10 6 per well) were seeded in a 12-well plate and differentiated overnight with 10 nM phorbol myristate acetate. Attached THP-1 cells were stimulated with 100 ng ml −1 lipopolysaccharide (Sigma) for 3 h and treated with DMSO, GSTO1 inhibitors or Glyburide (Enzo Life sciences) in serum-free media for 1.5 h followed by addition of 5 mM ATP (Sigma) for 30 min. Supernatant media was collected and precipitated using trichloroacetic acid. Cell fraction was collected and processed as described above. A unit of 40 μg of protein lysate was incubated with SDS sample buffer for 5 min at 90 °C, resolved on a 10% polyacrylamide gel and electroblotted on a polyvinylidene difluoride membrane. Membranes were blocked in 5% non-fat milk in Tris-buffered saline with 0.1% Tween-20 (TBST) for 1 h at room temperature and incubated overnight with primary antibodies at dilutions specified in Supplementary Table 26 . Subsequently, the membranes were washed with TBST and incubated with appropriate horseradish peroxidase-linked secondary antibodies for 2 h at room temperature followed by further washing with TBST. The immunoblots were visualized using ECL Western blotting substrate (Pierce Biotechnology) on a Chemidoc XRS imager (Bio Rad) or using Dylight 800-conjugated secondary antibodies (Thermo Fisher Scientific, Rockford, IL) on an Odyssey Imaging Systems (LI-COR Biosciences, Lincoln, NE). Band intensities were quantified using Image J software. Uncropped images of key western blots are presented in Supplementary Figs 25 and 26 . Bru-seq nascent RNA profiling HCT116 cells (4 × 10 6 ) were treated with siGSTO1 (10 nM), DMSO or C1-14 (10 μM) for 4 h or with C1-27 (1 μM) for 4 and 24 h. Nascent RNA was labelled, isolated and processed according to previously published protocol [27] , [57] . Pathway analysis GSTO1 Bru-Seq data set was filtered using the cutoff value of gene size >300 bp and mean reads per kilobase per million mapped reads (RPKM)>0.5, and a total of 8,072 genes in C1-27 4 h treatment, 8,324 genes in C1-27 24 h treatment, 8,172 genes in C1-14 4 h treatment and 8,962 genes in GSTO1 siRNA treatment groups were ranked based on fold change values versus control (DMSO) ( Supplementary Data Set 1 ). Shown in Supplementary Tables 10 and 11 and Supplementary Tables 14–19 are top 20 up- and downregulated genes in response to siRNA and drug treatments. The data set was analysed using the DAVID, ingenuity pathway analysis (IPA) and GSEA for pathway identification. DAVID ( http://david.abcc.ncifcrf.gov/home.jsp ) functional annotation analysis [28] , [58] was performed on the list of up- and downregulated genes with a fold change ≥1.4. Only those terms that reported a P value of ≤0.05 and count number ≥4 genes were selected for analysis. Pathway analysis of siGSTO1 Bru-Seq data was also performed using IPA (Ingenuity Systems, Inc., Redwood City, CA) with genes showing fold change ≥2. Data sets with nearly 250 genes containing the gene identifiers and fold changes were uploaded to the IPA web-based application and each gene identifier was mapped to its corresponding gene object in the ingenuity pathways knowledge base. Finally, the biological function genes were ordered by P value of significance and maximum number of genes in the pathway. Bru-Seq data were further analysed using GSEA for exploring the mechanism of cellular action of GSTO1 and its inhibitor. A pre-ranked gene list of the Bru-Seq data set was submitted to GSEA, and enrichment analysis was done based on the Kolmogorov–Smirnov statistic [59] , [60] . GSEA is a knowledge-based approach for interpreting genomic profiles based on the gene sets. For each gene set, the ES (enrichment score) was normalized to account for differences in gene set size and the false discovery rate relative to the normalized enrichment score values was calculated. Supplementary Tables 12 and 13 and Supplementary Tables 20–24 show the top GSEA gene sets for the up- and downregulated genes in siGSTO1 and drug treatment Bru-Seq data sets. In vivo efficacy studies In the pilot study, HCT116 cells (1 × 10 6 ) in exponential phase were injected subcutaneouslyinto the left flank of 8- to 10-week-old female nude mice (25–30 g; Simonsen laboratories, Gilroy, CA). The perpendicular diameters of the tumours were measured three times weekly using standard calipers and tumour volumes were calculated using the formula: 0.5 × D × d 2 , where D and d were the longest and shortest perpendicular diameters, respectively. Tumours were allowed to grow to a volume of 50 mm 3 and mice were randomized into control ( n =5) and C1-27 ( n =3) treatment groups. C1-27 dissolved in peanut oil was administered intraperitoneally (20 mg kg −1 per day) for the first 2 weeks on a 5 days on/2 days off schedule. The dose was then increased to 25 mg kg −1 per day for the next 23 days and further escalated by 5 mg kg −1 per day to a final dose of 45 mg kg −1 for the remaining duration of treatment. Tumour volumes and body weights were measured three times weekly to monitor tumour burden and weight loss during treatment. At the end of the experiment, animals were killed and tumour, kidney and liver were collected, fixed and paraffin-embedded for histology. The animal experiments were done in accordance with protocols approved by the University of Southern California Institutional Animal Care and Use Committee. For the colorectal cancer PDX study, female NCR nude mice (CrTac:NCr- Foxn1 nu from Taconic) were implanted subcutaneously with low-passage KRAS-mutant CRM 13–180 tumour fragments ( ∼ 30 mg) into the region of the right axilla. The CRM 13–180 PDX model was provided by the laboratory of Dr Judith Leopold (University of Michigan) [61] . Mice were randomized into treatment groups ( n =5) and treatments initiated when tumours reached ∼ 100 mg. C1-27 , SC-144 and As 2 O 3 were administered intraperitoneally in a fixed volume of 100 μl, on a 5 days on/2 days off schedule. L-OHP was administered intraperitoneally in a fixed volume of 100 μl once a week. Subcutaneous tumour volume and body weights were measured three times a week. Tumour volumes were calculated by measuring two perpendicular diameters with calipers and using the formula: tumour volume=(length × width 2 )/2. Mice were treated as indicated until the mean tumour burden in the vehicle control group reached ∼ 1,000 mg. Mice received a total of four cycles of treatment. % T / C was calculated by dividing the median treated tumour weight by the median control tumour weight and multiplying by 100 on the last day of treatment. Tumour growth delay ( T − C ) was calculated by subtracting the median time to reach evaluation size (750 mg) of the treated group by the median time to evaluation size of the control group. All procedures related to the handling, care and treatment of animals were conducted in accordance with University of Michigan’s Committee on the Use and Care of Animals guidelines. The investigators were not blinded in either study. Statistical analysis Data are presented as mean of at least three independent experiments and error bars denote s.e.m. or s.d. as indicated. Statistical analysis was done using Prism 7.0 (Graphpad software). Single comparisons were performed by two-sided Student’s t -test assuming unequal variance. Multiple comparisons were analysed using one-way analysis of variance or two-way analysis of variance followed by Dunnett’s post hoc test. P values at α =0.05 are reported (* P <0.05, ** P <0.01, *** P <0.001 and **** P <0.0001). For the PDX efficacy study, a sample size of five animals per treatment group was estimated to provide more than 80% power using two-sided P <0.05 criterion. Data availability The coordinates for GSTO1 inhibitor complexes have been deposited with the PDB: C1-27 (4YQM); C1-31 (4YQU) and C4-10 (4YQV). The Bru-Seq data discussed in this publication have been deposited in the NCBI Gene Expression Omnibus and are accessible through the GEO series accession number GSE85899 . All relevant data that support the findings of this study are available within the article and its Supplementary Information , or from the corresponding author on request. How to cite this article: Ramkumar, K. et al . Mechanistic evaluation and transcriptional signature of a glutathione S -transferase omega 1 inhibitor. Nat. Commun. 7, 13084 doi: 10.1038/ncomms13084 (2016).